Direct dynamic imaging of non-adiabatic spin torque effects Spin-transfer torques offer great promise for the development of spin-based devices. The effects of spin-transfer torques are typically analysed in terms of adiabatic and non-adiabatic contributions. Currently, a comprehensive interpretation of the non-adiabatic term remains elusive, with suggestions that it may arise from universal effects related to dissipation processes in spin dynamics, while other studies indicate a strong influence from the symmetry of magnetization gradients. Here we show that enhanced magnetic imaging under dynamic excitation can be used to differentiate between non-adiabatic spin-torque and extraneous influences. We combine Lorentz microscopy with gigahertz excitations to map the orbit of a magnetic vortex core with <5 nm resolution. Imaging of the gyrotropic motion reveals subtle changes in the ellipticity, amplitude and tilt of the orbit as the vortex is driven through resonance, providing a robust method to determine the non-adiabatic spin torque parameter β =0.15±0.02 with unprecedented precision, independent of external effects. In ferromagnets, the imbalance of spin populations of conduction electrons leads to a spin polarization of the electrical current, which transports angular momentum as well as electrical charge. To account for the interaction of the spin-polarized currents with the local magnetization, the phenomenological equation of motion—the Landau–Lifshitz–Gilbert (LLG) equation—is modified through the addition of two additional terms. With these terms, the LLG equation is: where the first two terms describe the precession of the magnetization, , about the effective field, , with α being the viscous damping parameter for spin dynamics and γ the gyromagnetic ratio. The third term describes the well-understood adiabatic processes related to the spin current, where , a velocity term, is related to the magnitude and direction of the current , as well as the degree of spin polarization, P (ref. 1 ). The final term relates to non-adiabatic processes whose magnitude is governed by β , the non-adiabatic parameter. The sources and origin of the non-adiabatic spin torque remain in question [1] , [2] and even its magnitude, essential to developing a working theory, is not clearly determined. Several studies determine that β ≈ α [3] , [4] , raising the intriguing notion that the non-adiabatic spin torque arises from universal processes related to dissipation. Alternatively, other reports indicate that β is considerably larger than α [4] , [5] , [6] . Remedying the incomplete understanding of non-adiabatic spin torque is of particular relevance because in current driven dynamics it governs domain wall velocity, which scales linearly with β below the Walker breakdown limit, where the domain wall begins to experience turbulent motion and mobility is greatly affected [6] , [7] , [8] . Thus, the development of new spin torque devices will be facilitated by a more complete understanding of the non-adiabatic torque [9] . Experimental constraints often make the direct measurement of β challenging. In nanowires, local structural variations and differing assumptions [10] , [11] have led to a range of reported values for β from β ≈ α to β >18 α , and recent results suggest that β should depend on the magnetization gradient in the sample [4] . Furthermore, to determine the relevant ratio β / α , these results assume values of α , which can vary greatly depending on the microstructure of patterned films. Simplified geometries such as disks and squares that exhibit a flux closure domain state (Landau state) can be used to circumvent some of the limitations of nanowire geometries. In a flux-closure or vortex state, the magnetization curls around in a clockwise (CW) or counter-CW (CCW) direction [12] , [13] , [14] . In square structures, the magnetization tends to follow the edges of the square to minimize the dipolar energy and diagonal Bloch walls form to reduce the quantum mechanical exchange energy. The centre, or core, of the vortex has a magnetization component orthogonal to the plane of the disk or square, the core polarity, p , which can point into or out of the plane ( p =±1). Electrical currents passing through magnetic vortex structures affect the domain distribution and the equilibrium position of a vortex core. It is difficult, however, to discriminate between the effects of spin-transfer torques and the Oersted fields in experiments involving electrical currents [15] , [16] , [17] , which complicates the determination of β . To date, the lowest reported relative error estimates of the non-adiabatic spin torque are based on X-ray imaging measurements of the position of a vortex core displaced by pulsed DC currents [6] . The Oersted contributions were cancelled out by reversing the chirality of the vortex. The relative uncertainties in the core positions, and hence in β , were almost 50% due to the limited spatial resolution of the technique. Furthermore, the vortex core is static in these measurements so it is susceptible to influences from strong local pinning [18] . Reducing the uncertainty in β would require a greater vortex core displacement, better spatial resolution, a dynamic approach or a combination of the above. Here, we implement a new technique that utilizes the unparalleled spatial resolution of electron microscopy and in situ resonant excitations to meet all of these requirements. By analysing the vortex core orbits, we are able to measure β with unprecedented precision. Measurement of gigahertz excitations with in situ microscopy To measure β with greater precision, we modified a customized, dedicated high-resolution Lorentz electron microscope (LEM, 1 nm spatial resolution and 30 ms time resolution in static magnetic imaging [19] ) by developing a new sample stage capable of applying high-frequency AC and pulsed excitations in situ ( Fig. 1a,b ). We utilize the gyrotropic dynamic mode of the Landau vortex structure in permalloy squares (typically 100 MHz–1 GHz) to quantify the various excitation effects ( Fig. 1c–e ). The vortex and its core can be considered as a composite quasiparticle and high-frequency magnetic fields and/or spin-polarized currents near the vortex gyrotropic resonance frequency excite elliptical motion of the vortex about its central equilibrium position. We image the steady-state motion of the vortex core as it is excited by an AC current oscillating at ~0.15–0.25 GHz, and directly observe the precession orbits of the vortex core. AC excitations near the gyrotropic resonance frequency result in the precession of the vortex core along an elliptical path that is largest at the resonance frequency ( Fig. 2a ). Since the period of the resonance of a vortex core is on the order of a nanosecond, we detect the trace of the orbit through time averaging over many cycles of the excitation, hence the images provide a record of the average orbit amplitude, ellipticity and tilt with high accuracy ( Fig. 2b ). 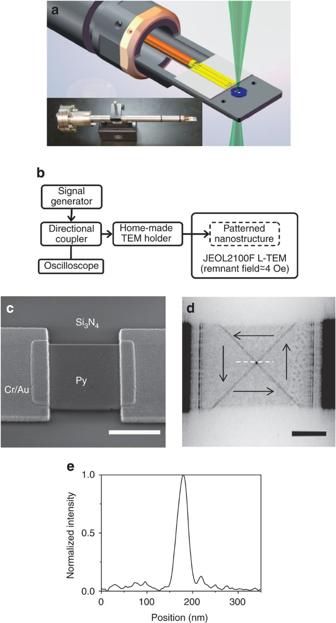Figure 1: Experimental setup and sample images. (a) Schematic layout of the TEM holder assembly with its actual image in the inset. A high-frequency signal is supplied externally through a coaxial cable (brown) and a copper waveguide (gold). The waveguide is wire bonded to gold contact pads on the silicon nitride Si3N4membrane (blue). (b) Connection diagram of thein situTEM excitation experiments. (c) A scanning electron microscopy image of the permalloy square and Cr/Au contact pads fabricated on the membranes. Scale bar, 1 μm. (d) Lorentz micrograph of the permalloy square showing the remnant state Landau domain structure. The arrows indicate the direction of the magnetization within each domain. Scale bar, 500 nm. (e) Linescan across the vortex core (indicated by the white line ind). The full width at half maximum of the vortex core is about 21 nm. The magnetic imaging resolution of the instrument is 1 nm, thus the accuracy of the vortex core positions in the experiments is not limited by the instrument. Figure 1: Experimental setup and sample images. ( a ) Schematic layout of the TEM holder assembly with its actual image in the inset. A high-frequency signal is supplied externally through a coaxial cable (brown) and a copper waveguide (gold). The waveguide is wire bonded to gold contact pads on the silicon nitride Si 3 N 4 membrane (blue). ( b ) Connection diagram of the in situ TEM excitation experiments. ( c ) A scanning electron microscopy image of the permalloy square and Cr/Au contact pads fabricated on the membranes. Scale bar, 1 μm. ( d ) Lorentz micrograph of the permalloy square showing the remnant state Landau domain structure. The arrows indicate the direction of the magnetization within each domain. Scale bar, 500 nm. ( e ) Linescan across the vortex core (indicated by the white line in d ). The full width at half maximum of the vortex core is about 21 nm. The magnetic imaging resolution of the instrument is 1 nm, thus the accuracy of the vortex core positions in the experiments is not limited by the instrument. 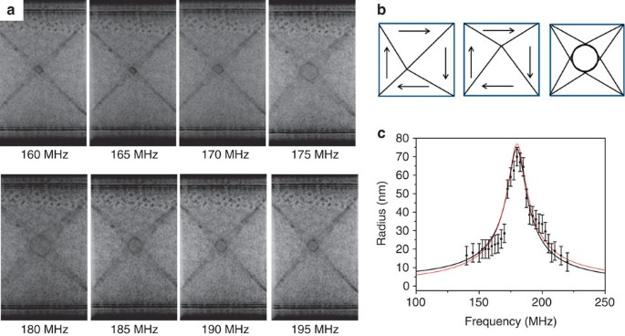Figure 2: Frequency dependence of vortex core precession orbit. (a) Lorentz micrographs of the vortex core precession orbit at various driving frequencies. An AC current was applied along the horizontal direction, with the current density maintained at 7.7×1010A m−2. (b) Schematic illustration of how the vortex motion leads to the patterns observed as images of the dynamic orbits. As the vortex precesses about the central equilibrium point, the domain walls of the Landau structure oscillate about their equilibrium positions, creating blurred domain contrast at their boundaries. The domains, which are pinned by each of the four corners of the spin structure and the vortex core, move with the vortex core. For clarity the image contrast was reversed. (c) Vortex core precession orbit amplitude versus driving frequency extracted from Lorentz micrographs. The AC current was applied along the horizontal (X) direction. The black dots show experimental data that represent an average of the maximum displacements of the core parallel and perpendicular to the current flow; the error bars reflect the uncertainty in fits of the observed orbits to an ellipse. The red and black curves are theoretical predictions based on the harmonic oscillator model. Full size image Figure 2: Frequency dependence of vortex core precession orbit. ( a ) Lorentz micrographs of the vortex core precession orbit at various driving frequencies. An AC current was applied along the horizontal direction, with the current density maintained at 7.7×10 10 A m −2 . ( b ) Schematic illustration of how the vortex motion leads to the patterns observed as images of the dynamic orbits. As the vortex precesses about the central equilibrium point, the domain walls of the Landau structure oscillate about their equilibrium positions, creating blurred domain contrast at their boundaries. The domains, which are pinned by each of the four corners of the spin structure and the vortex core, move with the vortex core. For clarity the image contrast was reversed. ( c ) Vortex core precession orbit amplitude versus driving frequency extracted from Lorentz micrographs. The AC current was applied along the horizontal (X) direction. The black dots show experimental data that represent an average of the maximum displacements of the core parallel and perpendicular to the current flow; the error bars reflect the uncertainty in fits of the observed orbits to an ellipse. The red and black curves are theoretical predictions based on the harmonic oscillator model. Full size image By carefully mapping the vortex trajectory for both vortex chiralities we discriminate between the effects of spin-torques and Oersted fields, permitting high-accuracy estimates for β . Figure 2 displays the response of the vortex core with CCW chirality to AC currents of varying frequency with a step size of 2.5 MHz. The theoretical amplitudes based on a harmonic oscillator model [15] , [17] , [20] match the experimental measurements well ( Fig. 2c ). The uncertainty is not only limited by the LEM resolution of the vortex core position, but is also due to local deviations from an elliptical orbit, possibly due to scattering from defects and grain boundaries. Spin torque effects on vortex core orbits Phenomenological descriptions of the vortex motion predict that the size of the orbit at resonance will depend not only on the magnitude of the excitation current but also on the chirality of the vortex if Oersted fields contribute to the excitation [15] , [17] . The Oersted field h o is perpendicular to the direction of current flow, which provides a force on the vortex core parallel or antiparallel to the current ( j o ) depending on the chirality and the nature of the current imbalance within the sample, typically attributed to higher current density near the top or bottom surface of the sample. The non-adiabatic spin torque acts in the same direction but is not sensitive to the chirality. Hence, it will either add to or partially cancel the effect of the Oersted field depending on the vortex chirality ( Fig. 3 ). The adiabatic spin torque, in contrast, acts perpendicular to both the Oersted field and the non-adiabatic spin torque and does not depend on chirality. 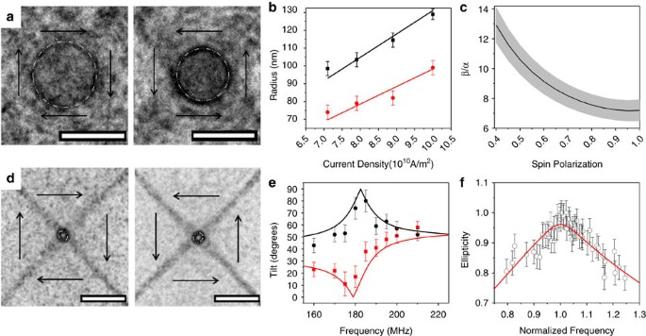Figure 3: Vortex core precession orbits due to the adiabatic, nonadiabatic and Oersted field contributions. (a) Experimental images of the vortex precession at resonance (170 MHz) at a current density of 1×1011A m−2. Clear differences in orbit amplitude are visible for vortices of CW (left) and CCW (right) chirality. The white dashed circles are a guide to the eye, and arrows indicate the sense of rotation of the vortex. Scale bar, 250 nm. (b) Orbit radius at resonance versus current density. The values are extracted from images of the orbit sizes at resonance. Red (black) points are from CCW (CW) vortices. A fit to these data (solid lines) yields a non-adiabatic parameterβ=(9.2±0.8)αand an Oersted field per unit current of 1.62×10−11±0.03×10−11Oe m2A−1(1.3 Oe for a current densityjoof 7.9×1010A m−2). (c) Experimentally determinedβ/αversus assumed spin polarization. The ratio ranges from ~7 to 13, showing a clear lower limit forβ. The error band corresponds to the uncertainty inβobtained from fits to the experimental amplitude versusjodata assuming a given value of spin polarization. (d) Off-resonance orbits at 200 MHz for vortices of (polarity=+1, CW) and (polarity=+1, CCW). The tilts of the orbit differ measurably, as predicted by theory. Black arrows indicate the sense of rotation of the vortex, while white dashed circles are superimposed on the vortex orbit to guide the eye. Scale bar, 250 nm. (e) Measured tilt from the current direction versus frequency for the same element atjo= 7.9×1010A m−2. The small shift in resonance frequency from that of a current density of 1×1011A m−2is due to Joule heating. (f) Ellipticity (defined as short axis/long axis) versus normalized frequency for CCW chiralities with a theoretical prediction superimposed (solid line). The characteristics of the vortex orbit at off-resonance frequencies are clearly observed, for the first time, through the direct imaging method. The experimental amplitudes, tilts, ellipticities and the associated uncertainties were determined by fitting the observed orbit to an ellipse. Figure 3: Vortex core precession orbits due to the adiabatic, nonadiabatic and Oersted field contributions. ( a ) Experimental images of the vortex precession at resonance (170 MHz) at a current density of 1×10 11 A m −2 . Clear differences in orbit amplitude are visible for vortices of CW (left) and CCW (right) chirality. The white dashed circles are a guide to the eye, and arrows indicate the sense of rotation of the vortex. Scale bar, 250 nm. ( b ) Orbit radius at resonance versus current density. The values are extracted from images of the orbit sizes at resonance. Red (black) points are from CCW (CW) vortices. A fit to these data (solid lines) yields a non-adiabatic parameter β =(9.2±0.8) α and an Oersted field per unit current of 1.62×10 −11 ±0.03×10 −11 Oe m 2 A −1 (1.3 Oe for a current density j o of 7.9×10 10 A m −2 ). ( c ) Experimentally determined β / α versus assumed spin polarization. The ratio ranges from ~7 to 13, showing a clear lower limit for β . The error band corresponds to the uncertainty in β obtained from fits to the experimental amplitude versus j o data assuming a given value of spin polarization. ( d ) Off-resonance orbits at 200 MHz for vortices of (polarity=+1, CW) and (polarity=+1, CCW). The tilts of the orbit differ measurably, as predicted by theory. Black arrows indicate the sense of rotation of the vortex, while white dashed circles are superimposed on the vortex orbit to guide the eye. Scale bar, 250 nm. ( e ) Measured tilt from the current direction versus frequency for the same element at j o = 7.9×10 10 A m −2 . The small shift in resonance frequency from that of a current density of 1×10 11 A m −2 is due to Joule heating. ( f ) Ellipticity (defined as short axis/long axis) versus normalized frequency for CCW chiralities with a theoretical prediction superimposed (solid line). The characteristics of the vortex orbit at off-resonance frequencies are clearly observed, for the first time, through the direct imaging method. The experimental amplitudes, tilts, ellipticities and the associated uncertainties were determined by fitting the observed orbit to an ellipse. Full size image At resonance, we find that the amplitude of the vortex core orbit is larger for a CW vortex as compared with a CCW vortex ( Fig. 3a,b ). A difference in orbit amplitudes for the different chiralities, A CW and A CCW , is a direct indication that both the Oersted field, h o , and the nonadiabatic spin torque effects are nonzero as , which follows from Krüger et al . [15] The larger CW orbits could indicate that there is a greater current flow along the bottom of the structure; however, numerical calculations favour a uniform current density across the thickness and reveal that the magnitude and direction of the Oersted field in these experiments is consistent with magnetic fields produced by the vertical flow of current at the contact pads. The constant of proportionality in the above relation depends only on measurable or known experimental parameters, known physical constants and parameters that can be extracted easily from micromagnetic simulations (see Methods for details). The sum of the squared amplitudes is approximately , where C 1 and C 2 are again constants that depend on parameters that are reliably know, which provides a means to estimate h o independent of β . Hence, the measurements of the orbit amplitudes for both chiralities and as a function of frequency allow for the unambiguous determination of β and α , respectively. In addition, we observe, for the first time, the tilting and ellipticity of the vortex core orbit at off-resonance frequencies, also in agreement with theory ( Fig. 3d–f ). At and near resonance the orbit is nearly circular. As the frequency moves off resonance, the ellipticity and the normalized frequency follow an almost linear relationship ( Fig. 3f ), as predicted by theory. The orbital tilts are sensitive to the relative magnitudes of all three driving contributions: adiabatic, non-adiabatic and Oersted. Hence, mapping the tilt angle with respect to frequency may allow the additional determination of the degree of spin polarization, P , though in practice, local pinning effects can influence low-amplitude oscillations and may complicate the interpretation of P [18] , [21] . Full micromagnetic simulations of the driven dynamics ( Fig. 4 ) were conducted, and compared with driven vortex core trajectories calculated using a simplified harmonic-oscillator theory [15] . They are in good agreement with each other, hence the analytic theory can be used to fit the experimental results to obtain α , β and h o . At resonance, the core trajectories are the largest and the shape is close to circular. Although the chirality greatly affects the amplitudes of the orbit, as seen in Fig. 4c,f , the results for each chirality compare favourably with our high-resolution dynamic images ( Fig. 3a ). Off resonance, the core trajectories are tilted and the tilt angles vary as a function of β , h o , P and frequency. For purely field-driven simulations, the core trajectories are almost parallel and perpendicular to the x axis above and below resonance, respectively ( Fig. 4e,g , insets). The amplitudes and tilts of the trajectories are both sensitive to the magnitude of the non-adiabatic spin torque; however, the former provide the most reliable means to determine β . 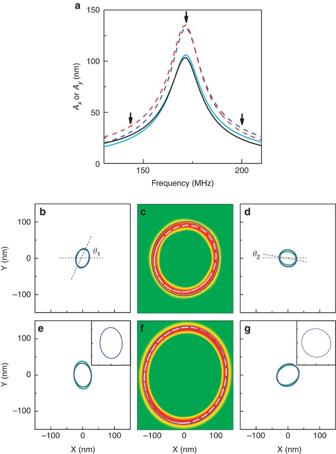Figure 4: Micromagnetic simulations and numerical calculations of the driven oscillations of a magnetic vortex in a permalloy square. (a) Theoretical predictions of the core amplitude,AxandAy, along and perpendicular to the direction of current flow, respectively, as a function of the frequency of the driving AC current for CW (solid lines) and CCW (dashed lines) vortex chiralities. BothAx(blue and cyan) andAy(red and black) are shown for both chiralities. Combined spin torque and Oersted effects were considered with an Oersted fieldho=1.7 Oe (corresponding to greater current flow along the top of the structure), current densityjo=7.7×1010A m−2, dampingα=0.016, spin polarizationP=0.6 and non-adiabatic parameterβ=10α. Arrows indicate the frequencies for which calculated trajectories are shown. (b–g) The theoretically predicted core trajectories at selected frequencies, below resonance at 140 MHz (b,e), at resonance (c,f), and above resonance at 200 MHz (d,g), for both CW (top,b–d) and CCW (bottom,e–g) chiralities for positive vortex polarity (blue lines). Trajectories from micromagnetic simulations (green lines) are superimposed. Differences in the tilt of the trajectory off resonance are shown for the CW orbits. The insets of (e) and (g) show the corresponding core trajectories for purely magnetic field-driven oscillations. At resonance (c,f) orbits are shown using full 3D simulations (white line) in comparison with the analytical model (blue line). The thickness- and time-averagedz-component of the magnetization is shown in the color plot; the red orbit shows the path of the vortex core. A 2×2 μm, 50-nm-thick permalloy square was used in the calculations. Figure 4: Micromagnetic simulations and numerical calculations of the driven oscillations of a magnetic vortex in a permalloy square. ( a ) Theoretical predictions of the core amplitude, A x and A y , along and perpendicular to the direction of current flow, respectively, as a function of the frequency of the driving AC current for CW (solid lines) and CCW (dashed lines) vortex chiralities. Both A x (blue and cyan) and A y (red and black) are shown for both chiralities. Combined spin torque and Oersted effects were considered with an Oersted field h o =1.7 Oe (corresponding to greater current flow along the top of the structure), current density j o =7.7×10 10 A m −2 , damping α =0.016, spin polarization P =0.6 and non-adiabatic parameter β =10 α . Arrows indicate the frequencies for which calculated trajectories are shown. ( b – g ) The theoretically predicted core trajectories at selected frequencies, below resonance at 140 MHz ( b , e ), at resonance ( c , f ), and above resonance at 200 MHz ( d , g ), for both CW (top, b – d ) and CCW (bottom, e – g ) chiralities for positive vortex polarity (blue lines). Trajectories from micromagnetic simulations (green lines) are superimposed. Differences in the tilt of the trajectory off resonance are shown for the CW orbits. The insets of ( e ) and ( g ) show the corresponding core trajectories for purely magnetic field-driven oscillations. At resonance ( c , f ) orbits are shown using full 3D simulations (white line) in comparison with the analytical model (blue line). The thickness- and time-averaged z -component of the magnetization is shown in the color plot; the red orbit shows the path of the vortex core. A 2×2 μm, 50-nm-thick permalloy square was used in the calculations. Full size image Determination of β We carefully tuned the frequency in the experiments until the maximum core trajectory is observed and fit the resonant amplitudes as a function of current for both chiralities to obtain β . Currents were chosen such that the maximum vortex core displacements were only 6.5% of the disc width to prevent anharmonic contributions to the motion, but to still maintain large enough displacements to minimize the pinning effects that are present for static or weakly driven excitations [18] , [21] . This represents one of the key advantages of our approach, as pinning can lead to large errors [6] . We perform two independent fits, one to the amplitude as a function of frequency, which provides α independent of β . Then, we fit the amplitude at resonance as a function of current for both chiralities to obtain β . The slopes of A CCW 2 − A CW 2 versus j o and A CCW 2 + A CW 2 versus j o 2 yield estimates for β and h o , which were then refined using nonlinear fits to the full theory, as described in more detail in the Methods. The only external input into the fits is the degree of spin polarization. By fitting the experimental observations, we determine that the Gilbert damping (measured specifically for this sample) is α =0.016±0.001 ( Fig. 2c ) and β =0.15±0.02=(9.2±0.8) α . These fits assume a spin polarization value of P =0.6 (ref. 22 ). The value obtained for β is comparable to that obtained from the depinning of vortex walls in nanowires, and an order of magnitude larger than that found in transverse walls [3] , [4] . Taking into consideration the full range of reported P values, we may assign a minimum bound of β =7 α ( Fig. 3c ) [4] , [23] (see Supplementary Discussion for additional detail). By combining high-resolution measurements of the vortex core trajectory with analytic and micromagnetic simulations, we have quantified the spin torque and Oersted contributions to the vortex dynamics with unprecedented precision, determining β/α =9.2 with an estimated uncertainty that is approximately a 300% improvement over previous works [6] . The detailed measurement of the non-adiabatic spin torque parameter will allow close comparison with theoretical investigations on the origins of β . Indeed, we also observed, for the first time, the off-resonance effects of non-adiabatic spin torques. The high value of β determined here is attractive for spintronic applications, as it implies high domain wall velocities can be obtained, which would facilitate the development of fast and low-power technologies [8] . Moreover, the capabilities of high-resolution imaging of dynamic processes with LEM point to a new paradigm in magnetic microscopy. The development may lead to innovative measurements such as spin polarization in vortex structures measured under AC excitations, and may impact several diverse fields within nanomagnetism. For example, the accuracy of recent measurements of static vortex shape and core trajectories in spin torque nano-oscillators [24] can be re-examined with the improved resolution of electron microscopy. Also, with advances in sensitivity, the time-averaged and high-resolution imaging technique can be extended to image spin wave patterns in magnonic crystals [25] , as well as real-space studies of nodal patterns in arrays of phase-locked spin torque nano-oscillators [26] acting as spin-wave point sources. Such capabilities will be of great value in developing these promising technologies for computation and communications applications. Experiment The home-made TEM specimen stage ( Fig. 1a ) was designed to deliver high-frequency electrical signals (0.1 MHz–1 GHz) into a sample region with minimal signal loss and waveform distortion. An external signal was transmitted from the outside signal generator to the stage by an ultra-high vacuum compatible coaxial cable with 50 Ω impedance. This microwave signal is then transmitted via a Cu coplanar waveguide patterned on a printed circuit board with the Cu waveguide wire bonded to the contact pads on the Si 3 N 4 membrane. Magnetic squares (2 μm×2 μm×50 nm) were fabricated on 100-nm-thick Si 3 N 4 electron transparent membranes using electron beam lithography followed by the deposition of 50 nm of permalloy (calibrated within 1 nm). Cr/Au (5 nm/100 nm) striplines were fabricated and deposited using a similar method and connected by wire bonding to the coaxial cable. A backlayer of Cr (3 nm) was deposited on the other side of the membrane to help with heat dissipation. Signals were supplied externally to the TEM by an Agilent N5181A MXG analog signal generator (100–1,000 MHz, −110 to 13 dBm). The signal was sampled by a coaxial directional coupler (Mini-circuits, ZFDC-20-4L) and the waveform was monitored by a Tektronics TDS 3052C Oscilloscope. Experiments were carried out in a JEOL 2100F-LM microscope with a weakly excited long focal length pole-piece specifically designed for magnetic imaging, with a residual field <4 Oe out of the specimen plane. Contact resistance was inspected before TEM measurements using two-point probe. Before excitation, LEM images of the static Landau structure were analysed. It was found to exhibit a spin configuration of four equal sized triangular domains, corresponding to a traditional flux closure structure of a particular chirality, with the vortex core at the centre. Chirality is determined directly through Lorentz imaging, as it is highly sensitive to the direction of rotation of the local magnetization. The square shape was utilized owing to the existence of analytic models in which trajectories can be calculated without time consuming micromagnetic simulations and permalloy was used because extensive data on the materials have been compiled [22] . To switch the chirality, the sample was removed from the LEM column and a static magnetic field was applied in the plane of the sample. Orbit sizes, ellipticities, tilts and their associated uncertainties were determined by fitting the experimental images with an ellipse. Micromagnetic modelling Full micromagnetic simulations based on the extended LLG equations incorporating both adiabatic and non-adiabatic spin torque effects were conducted [27] and compared with the analytical models at selected frequencies to verify that the model provides an accurate description of the vortex dynamics for our sample parameters. Simulations of a square, 2,000×2,000×50 nm 3 , represented using cells of 4×4 nm, were conducted using materials parameters for permalloy: saturation magnetization M s =8.00×10 5 A m −2 , exchange constant A =1.3×10 −11 J m −1 and a gyromagnetic ratio of γ =1.76×10 11 Hz T −1 . We used a spin polarization value of P =0.6 (ref. 22 ), a damping parameter of α =0.016 and a nonadiabatic spin torque parameter of β =10 α . Simulations of free oscillations of the magnetic vortex core as a function of time were conducted after removing a DC magnetic field of 10 Oe and immediately after applying a 7.7-mA DC current ( Supplementary Fig. S1 ). The simulations were initialized using a relaxed vortex spin configurations obtained using a large damping parameter of 1 for fast convergence The oscillations follow damped sinusoidal motion X ( t )= A x e −Γ t sin( ω o t + φ ), where X is the core position, A x is the amplitude and φ is a phase factor. Fits to the oscillations yield the resonance frequency ω o /2 π =167 MHz, close to the experimentally measured average value of 172 MHz, and the decay parameter Γ=42.4 MHz for both the field- and current-driven simulations. Driven dynamic simulations were conducted for selected frequencies using a combined AC magnetic field and AC current of h o =1.7 Oe and j o =7.7×10 10 A m −2 . The values used for h o and β are higher than those that were ultimately established by fits to the experimental data, nevertheless they allow a comparison to be made between the simulations and the analytical theory. The driven dynamic simulations were run until steady-state motion of the vortex was observed (>20 periods). The free oscillation simulations were conducted using both 50 nm (2D (dimensional)) and 10 nm (3D) cells across the thickness and showed similar behaviour (2% change in resonance frequency, slight change in decay parameter, <2 nm shift in core position through the thickness). Owing to the computational expense of the driven simulations, Fig. 4 shows mainly 2D simulation results; the trajectories in Fig. 4c,f were extracted from full 3D simulations. Analysis The motion of a magnetic vortex is well described by Thiele's equation [20] , a phenomenological formula that uses a harmonic-oscillator-based approach to describe the vortex core motion X ( t )=( X ( t ), Y ( t )) as a function of time t . An extended version of the theory that includes both adiabatic and non-adiabatic spin torque contributions is given in Krüger et al . [15] as where is the AC driving current, and b j = Pμ B /| e | M s is a coupling constant for the current, where μ B is the Bohr magneton, and e is the charge of an electron. The equation also involves the vortex gyrovector G o =− p | G o |=−2 πpTM s / γ , where T is the thickness of the magnetic structure, and the vortex energy profile W ( X ) that includes a harmonic-like dipolar energy term that provides a restoring force and the Zeeman energy that describes the coupling of the vortex to the driving magnetic field. D Γ and D o are damping parameters that should be similar in magnitude and constant for a given sample geometry and material [28] . The steady-state solution for the vortex core motion for combined spin torque and field-driven motion is given by equation (17) in the Supplementary materials of Krüger et al . [15] : here ω is the driving frequency, , l is the lateral width of the square and c is the vortex chirality. The sinusoidal current and Oersted field act along the x axis and y axis, respectively. The decay parameter Γ replaces the damping parameter D Γ in the above equation where the two are linked by the relation D Γ =Γ| G o |/( ω o α ). The damping parameters D Γ and D o are determined from fits to simulations of free oscillations of the magnetic vortex, which yield D Γ / G o = D o / G o =2.52 for our experimental geometry. The above model yields solutions for the vortex core motion that are, in general, elliptical in shape. At resonance, it follows from equation (2) that the difference of the core amplitudes squared for the two chiralities is approximately . The difference of the squared amplitudes is proportional to β but it also depends on h o . The average amplitude squared, however, is approximately . Hence, the sum and difference of the resonant amplitudes squared can be used together to determine both h o and β . More accurate values for β and h o were obtained by fitting the amplitude data with the full theory (equation 2) using a nonlinear least squares routine. We perform two independent fits to the experimental data to extract first α , and second h o and β . As mentioned above, the ratio D / G =2.52 was extracted from the 3D micromagnetic simulations of the free oscillations. We also used the simulations to obtain a refined estimate of the relationship between the orbit amplitude and the magnetization. The model above assumes triangular domains for the magnetization, which predicts X = l ( M y/ M s ). Fits to the micromagnetic simulation results ( Supplementary Fig. S1c ) yield l =1,900 nm, slightly lower than the predicted value. This correction has been applied to the fits to the experimental data ( Fig. 3 ) and the calculated trajectories ( Fig. 4 ). All other parameters are known or measured. We first use the theoretical model to fit the experimental measurements of the orbit amplitude versus frequency to obtain the damping constant α . This fit returns the same value, α =0.016±0.001, independent of the choice of β and h o . Finally, we use the theory along with the parameters determined above ( α , D o / G o , D Γ/ G o , and l ) to fit the experimental measurements of the average orbit amplitude at resonance as a function of j o to obtain β and h o . In this second fit, β and h o are the only remaining unknown parameters. They are independent of one another and hence uniquely determined. How to cite this article: Pollard, S.D. et al . Direct dynamic imaging of non-adiabatic spin torque effects. Nat. Commun. 3:1028 doi: 10.1038/ncomms2025 (2012).